Microelectromechanical Maltese-cross metamaterial with tunable terahertz anisotropy Dichroic polarizers and waveplates exploiting anisotropic materials have vast applications in displays and numerous optical components, such as filters, beamsplitters and isolators. Artificial anisotropic media were recently suggested for the realization of negative refraction, cloaking, hyperlenses, and controlling luminescence. However, extending these applications into the terahertz domain is hampered by a lack of natural anisotropic media, while artificial metamaterials offer a strong engineered anisotropic response. Here we demonstrate a terahertz metamaterial with anisotropy tunable from positive to negative values. It is based on the Maltese-cross pattern, where anisotropy is induced by breaking the four-fold symmetry of the cross by displacing one of its beams. The symmetry breaking permits the excitation of a Fano mode active for one of the polarization eigenstates controlled by actuators using microelectromechanical systems. The metamaterial offers new opportunities for the development of terahertz variable waveplates, tunable filters and polarimetry. Recently, in addition to traditional applications in optical filters and polarization components, anisotropic media was suggested for the realization of various important novel ideas, including negative refraction [1] , [2] , cloaking [3] , [4] , hyperlenses [5] , [6] , and controlling luminescence [7] , [8] . However, although asymmetries of crystalline lattices and their constiuent molecules often result in optical anisotropy of natural materials, it is very difficult to find the required values of optical anisotropy for a prescribed wavelength, in particular in the far-infrared and terahertz parts of the spectrum. On the contrary, metamaterials can be rationally designed to achieve optical anisotropy [9] , [10] , [11] , [12] , [13] , [14] , [15] , [16] , [17] , [18] , [19] that can also be altered by changing the refractive index of the surrounding medium [20] , [21] , [22] , [23] or by emplying electrical or thermal effects in liquid crystals [24] , [25] . At the same time, substantial progress has been possible in developing metamaterials with unit cells reconfigurable with micro-actuators [26] , [27] , [28] , [29] , [30] , [31] , [32] , [33] , [34] , [35] . Here we report the active control of anisotropy in the terahertz spectral region in a metamaterial array of Maltese crosses driven by micro-actuators. By breaking the four-fold symmetry of the cross, we show that it is possible to tune linear birefringence and dichroism of the array between the positive and negative values. Tunable metamaterial with Maltese-cross-shaped unit cells The metamaterial presented here is a two-dimensional square-lattice array of Maltese crosses with unit cell of 28 × 28 μm 2 ( Fig. 1a ). It is designed to operate in the terahertz range of the spectrum and was characterized from 1 to 5 THz. The micro-actuator framework allowed for a simultaneous reconfiguration of all unit cells in the array. This was achieved by manufacturing one of the trapezoid metal beams in each unit cell on a movable actuated silicon framework (coloured green in Fig. 1 ). Three other beams of the Maltese cross are fixed to the substrate (blue in Fig. 1 ). The movable beam of the cross can be shifted away from the cross centre to a distance S up to half of its length. 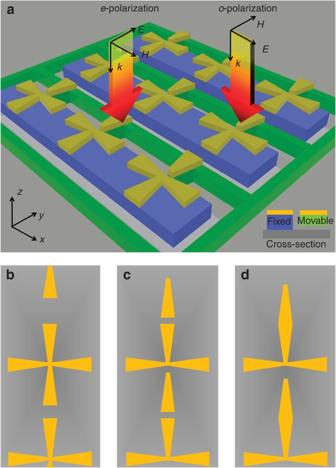Figure 1: Schematics of the micromachined Maltese-cross metamaterial. (a) The unit cell consists of four trapezoid metal stripes, one of which is located on the movable frames connected with the comb-drive actuator (green). The rest of the unit cell is located on the isolated islands (blue) fixed on the substrate. Inset shows the cross view of the unit cell. (b,c,d) The evolution of the unit cell when the movable trapezoid is shifted with the distanceS=0, 2.5 and 5 μm, respectively, is shown. Figure 1b–d shows the unit cell for S =0, 2.5 and 5 μm, respectively. The metamaterial sample with an overall size of approximately 1 cm 2 (400 × 400 unit cells) was fabricated on a silicon-on-insulator wafer as shown in Fig. 2a . 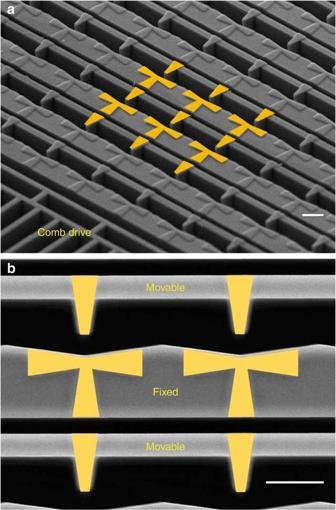Figure 2: Scanning electron microscopy image of the micromachined tunable metamaterial. (a) Overview of the unit cell array and comb drive. (b) Zoomed view of the Maltese-cross-shaped unit cell (the metal part is highlighted with false colour). The scale bars are 10 μm. Figure 2b shows a close-up view of the unit cells, which are formed by patterning a 0.5-μm thick evaporated aluminium layer. The design parameters are shown in Supplementary Fig. S1 . Figure 1: Schematics of the micromachined Maltese-cross metamaterial. ( a ) The unit cell consists of four trapezoid metal stripes, one of which is located on the movable frames connected with the comb-drive actuator (green). The rest of the unit cell is located on the isolated islands (blue) fixed on the substrate. Inset shows the cross view of the unit cell. ( b , c , d ) The evolution of the unit cell when the movable trapezoid is shifted with the distance S =0, 2.5 and 5 μm, respectively, is shown. Full size image Figure 2: Scanning electron microscopy image of the micromachined tunable metamaterial. ( a ) Overview of the unit cell array and comb drive. ( b ) Zoomed view of the Maltese-cross-shaped unit cell (the metal part is highlighted with false colour). The scale bars are 10 μm. Full size image When the four metal trapezoid beams are arranged into the pattern of the Maltese cross that has a four-fold symmetry axis, the metamaterial array exhibits no birefringence for normally incident radiation. On the contrary, when the four-fold symmetry of the design is broken by moving one of the beams off-centre, the metamaterial retains a plane of symmetry and becomes birefringent for normally incident light. We define the extraordinary polarization ( e -polarization) and ordinary polarization ( o -polarization) of this metamaterial with reference to the mirror symmetry axis of the pattern ( Supplementary Fig. S1 ). The e -polarization is parallel to the line of symmetry, whereas the o -polarization is perpendicular to it. Experimental results on birefringence and dichroism Optical anisotropy of the sample is completely characterized by its linear birefringence, and dichroism can be derived from its polarization-sensitive transmission and phase retardation spectra. The transmission spectra were measured by using an optical pump-terahertz probe (OPTP) system for different levels of asymmetry of the Maltese cross ( Fig. 3 ). The experimental setup and data analysis approaches are discussed in the Methods and Supplementary Figs S2–S6 . These measurements show that indeed at zero displacement S , when the cross has a four-fold symmetry, the metamaterial shows no dichroism: the recorded absorption spectra for both the o - and e - polarizations are nearly identical with the transmission peaks located at approximately 3.11 and 3.14 THz, respectively. Displacement of one of the beams of the cross is signified by a strong modification of the transmission spectrum for the e -polarization, including the appearance of a new transmission peak >4 THz, whereas the transmission spectrum for the o -polarization remains practically unchanged. The transmission peak moves from 3.11 to 2.73 THz, when the beam displacement changes from S =0 to 5 μm. See more detail on variation of dichroism in Supplementary Figs S7–S9 . 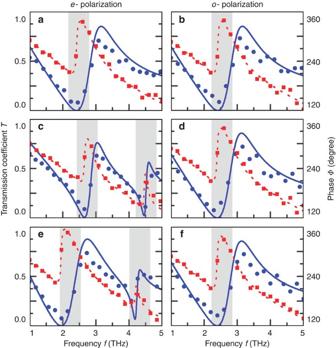Figure 3: Measured transmission and phase spectra of the Maltese-cross metamaterial. The first and second columns represente- ando-polarized incident light, respectively. The blue solid lines and circular symbols show the numerical and experimental analyses of the transmission, respectively. The red dotted line and square symbols show the numerical and experimental analyses of the phase, respectively. The first, second and third rows show the spectra, when the shift distance isS=0 μm (a,b), 2.5 μm (c,d) and 5 μm (e,f), respectively. Rapid phase changes in the frequency domain are highlighted in gray. Figure 3: Measured transmission and phase spectra of the Maltese-cross metamaterial. The first and second columns represent e - and o -polarized incident light, respectively. The blue solid lines and circular symbols show the numerical and experimental analyses of the transmission, respectively. The red dotted line and square symbols show the numerical and experimental analyses of the phase, respectively. The first, second and third rows show the spectra, when the shift distance is S =0 μm ( a , b ), 2.5 μm ( c , d ) and 5 μm ( e , f ), respectively. Rapid phase changes in the frequency domain are highlighted in gray. Full size image Anisotropy of the metamaterial was also characterized by measuring the differential phase retardation Δ Φ = Φ e − Φ o and transmitted power ratio T e / T o for e - and o -polarized waves as functions of S (see Fig. 4 ). Large phase changes of the transmission are observed at the frequency regions highlighted by grey colour as shown in Fig. 3a–f , where the transmission powers are bounced from the minimum to the maximum. Here the incident frequencies are fixed at 3.0 and 4.6 THz, which are the transmission peak frequencies at S =2.5 μm. However, large tunability of optical anisotropy of both 3.0- and 4.6-THz incidence is observed either at 0 μm< S <1 μm or 4 μm< S <5 μm, when the gap between the movable beam and the fixed part is significantly small as shown in Fig. 4 . The optical anisotropy is changed abruptly, when the movable beam is disconnected from the fixed ones. For f =3 THz, the phase difference is not sensitive to the shift distance S in the range from 1 to 4 μm. At the same time, the anisotropy monotonically increased at the high frequency of f =4.6 THz as shown in Fig. 4b . The anisotropy is more sensitive to the shift distance S at 4.6 THz than that at 3.0 THz. The tuning of the anisotropy depends on the variation of the dipole resonance mode of the Maltese cross, which is shown in Fig. 5 . The transmission ratio variation ( T e / T o ) is approximately 1 and 1.2 for f =3 and 4.6 THz, respectively. The effective refractive index of the Maltese-cross metamaterials is derived by fitting the measured transmission spectra with the Fresnel equations [36] . The differences between the effective refractive indices of o - and e -polarized incidence are shown in Supplementary Fig. S9 , which shows the same trend as the phase differences shown in Fig. 4 . 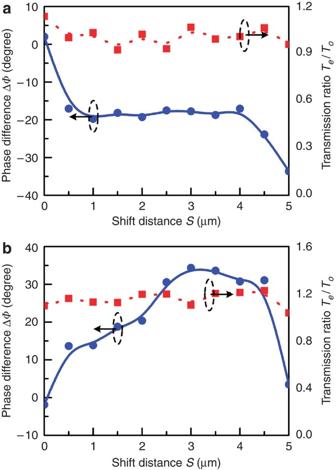Figure 4: Measured phase difference and transmitted power ratio betweene- ando-polarized light as functions of the shift distance. (a,b) The measurement results when the incident frequency is fixed at 3.0 and 4.6 THz, respectively, are shown. The measurement results and their trend are shown by the symbols and lines, respectively. Figure 4: Measured phase difference and transmitted power ratio between e - and o -polarized light as functions of the shift distance. ( a , b ) The measurement results when the incident frequency is fixed at 3.0 and 4.6 THz, respectively, are shown. The measurement results and their trend are shown by the symbols and lines, respectively. 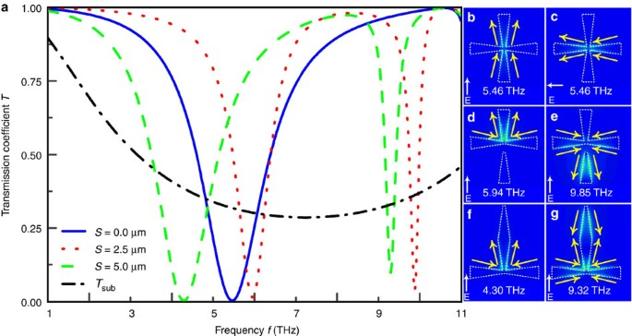Figure 5: Transmission spectra at different shift distance and surface current contour maps of the Maltese cross without substrate. (a) The solid, dotted and dashed lines represent the transmission spectra of the Maltese cross when the shift distanceSis 0, 2.5 and 5 μm, respectively. The transmission of the 3-μm substrate is represented by the black dash dotted line. (b–g) The contour maps show surface currents under excitation by different frequencies of light. The lighter colour shows the high density of surface current, and the arrows show the surface current flux direction. The direction of the incident electric field is marked with the white arrow at the lower left corner. The direction of the surface current is marked with the yellow arrow. Full size image Figure 5: Transmission spectra at different shift distance and surface current contour maps of the Maltese cross without substrate. ( a ) The solid, dotted and dashed lines represent the transmission spectra of the Maltese cross when the shift distance S is 0, 2.5 and 5 μm, respectively. The transmission of the 3-μm substrate is represented by the black dash dotted line. ( b – g ) The contour maps show surface currents under excitation by different frequencies of light. The lighter colour shows the high density of surface current, and the arrows show the surface current flux direction. The direction of the incident electric field is marked with the white arrow at the lower left corner. The direction of the surface current is marked with the yellow arrow. Full size image Origin of the tunable optical anisotropy The numerical analysis of the Maltese-cross structure without the substrate shows the dipole resonances of the surface current as shown in Fig. 5b–g , which result in transmission dips in the spectra. For example, when S=2.5 μm, the dipole resonance at 5.94 and 9.85 THz ( Fig. 5a ) can be mapped to the two Fano resonance dips as shown in Fig. 3c . The existence of the substrate has two effects. One is shifting the resonance dips to low frequencies, which is due to the permittivity difference between air and silicon substrate [37] . The other effect is leading to Fano-type resonance profile, which is due to the coupling between the dipole resonance modes of the Maltese cross and the Fabry–Pérot mode of the substrate [38] . The resonance frequency shifts shown in Fig. 3a are mainly due to the resonance features of the Maltese-cross design. Because the influence of the substrate does not change with the reconfigurations of the cross, we can conclude that spectral changes observed with the movements of the beams are due to the changes in the dipole resonance of the cross pattern. When the Maltese cross has a four-fold symmetry, the surface current is resonant between two opposite beams of the Maltese cross, which are parallel to the incident electric field, as shown in Fig. 4b . The other two beams have trivial effect on the dipole resonance. Therefore, the shifting of the Maltese-cross beam has trivial effects on the resonance modes when the movable beam is perpendicular to the incident electric field ( o -polarization). Considering the e -polarized incidence, however, the changing of the symmetry has vital effects on the dipole resonance modes due to the structural change of the beams, where most of the induced surface currents are concentrated on. This explains the difference between e- and o -polarized incidence of the transmission spectra as a function of shift distance S , which is shown in Fig. 3 . The tuning of the anisotropy can also be explained by the change of the resonance mode of the Maltese cross when the movable beam is actuated. At low frequencies, the surface current cannot go to the movable beam, which is disconnected from the remaining parts of the Maltese cross. The surface current is mainly concentrated at the fixed beam parallel to the incident electric field. This beam is weakly coupled to the two perpendicular beams. Therefore, the change of the shift distance S has small effects on the resonance mode of the Maltese cross, which explains the small variation of the optical anisotropy, when S is in the range from 1 to 4 μm under 3.0-THz incidence ( Fig. 4a ). At high frequencies, the surface current is mainly concentrated at the movable beam and has a π phase difference from the incident electric field. Therefore, the surface current resonance is mainly induced by the capacitance coupling between the fixed and movable beams of the Maltese cross. This capacitance is a strong function of the shift distance S . Therefore, the resonance mode of the Maltese cross is a strong function of the shift distance S , which explains the rapid tuning of the anisotropy, when S is in the range from 1 to 4 μm under 4.6-THz incidence ( Fig. 4b ). There is an abrupt resonance mode change at both low and high frequencies when the movable beam is being disconnected from the fixed parts, which explains the abrupt anisotropy change observed either at 0 μm< S <1 μm or 4 μm< S <5 μm for both incident frequencies as shown in Fig. 4 . Insertion loss of the tunable metamaterial The insertion loss of the tunable metamaterial consists of three parts, the ohmic loss due to the electron resonance within the metal structure, the reflection and the scattering loss of the imperfect surface and edge. In the experiment, the total insertion loss can be measured by monitoring the output transmission versus the source. 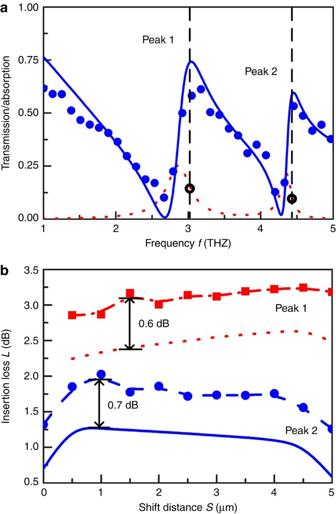Figure 6: Experimental and numerical analyses of the insertion loss for the reconfigurable metamaterial. (a) The transmission (blue solid line) and absorption (red dotted line) spectra under the shift distanceS=0.5 μm. The transmission peak and absorption peaks are staggered in the frequency domain. (b) The insertion losses of each transmission peak, when the shift distanceSranges from 0 to 5 μm. Peak 1 and Peak 2 refer to the transmission peaks at the low- and high-frequency regions, respectively. The lines and symbols represent the numerical and measured results, respectively. Figure 6a shows the transmission and absorption spectra under the shift distance S =0.5 μm. Peak 1 and Peak 2 represent the transmission peaks, when the shift distance S is in the range from 0 to 5 μm, at low- and high-frequency region, respectively. The transmission peak and absorption peaks are staggered in the frequency domain, which is similar at different shift distance S . Therefore, the ohmic loss is maintained under 12% at low-frequency region and 6% at high-frequency region. The ohmic losses of the transmission peaks under different shift distances S are shown in Supplementary Fig. S8 . The transmission peaks in high-frequency region have lower ohmic absorption because of the rapid decaying of the absorption profile at high-frequency region. The measured total insertion losses of the tunable metamaterial for Peak 1 and Peak 2 are shown in Fig. 6b . The symbols and lines show the experimental and numerical results, respectively. The differences of the experimental and numerical results are approximately 1 dB, which is due to the misalignment, surface roughness and edge scattering of the tunable metamaterial. Figure 6: Experimental and numerical analyses of the insertion loss for the reconfigurable metamaterial. ( a ) The transmission (blue solid line) and absorption (red dotted line) spectra under the shift distance S =0.5 μm. The transmission peak and absorption peaks are staggered in the frequency domain. ( b ) The insertion losses of each transmission peak, when the shift distance S ranges from 0 to 5 μm. Peak 1 and Peak 2 refer to the transmission peaks at the low- and high-frequency regions, respectively. The lines and symbols represent the numerical and measured results, respectively. Full size image The breaking of the Maltese-cross symmetry results in the splitting of the two parallel Maltese-cross beams and, subsequently, two different resonators, which can be excited by the e -polarized incidence. The breaking of the Maltese-cross symmetry splits and tunes the resonance modes of the e -polarized incidence but has minor effects on the o -polarized incidence with the electric field perpendicular to the mirror symmetry axis, which is unaltered during the tuning. The Maltese-cross metamaterial is tuned between positive anisotropy, negative anisotropy and isotropy states by actuators using microelectromechanical systems, which have promising applications such as waveplates, birefringent filters and light modulators. Fabrication processes The structures of the tunable metamaterial are fabricated on a silicon-on-insulator wafer by using the deep reactive ion etching processes [39] , [40] . Figure 2a shows the overview of the micromachined tunable metamaterial imaged by using the scanning electron microscopy. Two identical micromachined comb drive actuators driven by the electrostatic force are placed on both sides of the unit cell array. Each actuator provides bidirectional in-plane translation (along the x direction) following the actuation relationship Δ x = AV 2 , where Δ x is the displacement, V the actuation voltage and A =0.05 μm V −2 is the actuation coefficient. The displacement of the actuator can be monitored by using vertical microscopic system. The actuation coefficient A is derived by fitting the measured displacement–voltage curve. The actuation frequency can reach 10 kHz based on the dynamic measurement results of our previous work 40 . Figure 2b shows a close-up view of the unit cells. The micro-ring unit cells are formed by patterning a 0.5-μm thick evaporated aluminium layer on the top of the structure layer. The movable split rings are patterned on the central frame, which consists of many crossed narrow beams (2-μm width). The fixed split rings are patterned on the isolated anchors. Because each anchor encloses a larger area of the underlying oxide layer than the frame, it needs much longer time to remove all the oxide under the anchor than that under the frame. Therefore, the supporting frame is fully released and becomes freely movable, whereas the anchor remains fixed on the substrate by controlling the release time. Experimental setup Supplementary Figure S2 shows the experimental setup of the OPTP system used in the experiment. The terahertz probe pulse is generated by 35-fs pulses at centre wavelength of 800 nm with a repetition rate of 1 kHz by using the air-plasma technique. The spectral range of the terahertz pulse is from 0.3 to 8 THz, which is detected by free-space electro-optical (EO) sampling with a 0.3-mm thick <110> GaP crystal. The probe terahertz wave passes through the samples at normal incidence. The time domain terahertz signal is detected by the EO detector using a terahertz time-domain spectroscopy (TDS) delay system. It should be pointed out that the pump-probe system of the OPTP, which is highlighted as a red dashed line, is not used during the experiment because the Maltese-cross metamaterial is not tuned by laser pulses. Therefore, this OPTP system functions solely as a typical THz-TDS system in the experiment. The transmission spectra of both amplitude and phase, as shown in Supplementary Figs S5 and S6 , are derived by using the Fourier transform of the time domain signal from the EO detector and then normalized with the source spectra. In Fig. 3 , 20 equally spaced data points with the least mean-square error is chosen and compared with the simulation results. How to cite this article: Zhu, W. M. et al . Microelectromechanical Maltese-cross metamaterial with tunable terahertz anisotropy. Nat. Commun. 3:1274 doi: 10.1038/ncomms2285 (2012).